Pillararene incorporated metal–organic frameworks for supramolecular recognition and selective separation Crystalline frameworks containing incorporated flexible macrocycle units can afford new opportunities in molecular recognition and selective separation. However, such functionalized frameworks are difficult to prepare and challenging to characterize due to the flexible nature of macrocycles, which limits the development of macrocycle-based crystalline frameworks. Herein, we report the design and synthesis of a set of metal–organic frameworks (MOFs) containing pillar[5]arene units. The pillar[5]arene units were uniformly embedded in the periodic frameworks. Single crystal X-ray diffraction analysis revealed an interpenetrated network that appears to hinder the rotation of the pillar[5]arene repeating units in the frameworks, and it therefore resulted in the successful determination of the precise pillar[5]arene host structure in a MOF crystal. These MOFs can recognize paraquat and 1,2,4,5-tetracyanobenzene in solution and selectively remove trace pyridine from toluene with relative ease. The work presented here represents a critical step towards the synthesis of macrocycle-incorporated crystalline frameworks with well-defined structures and functional utility. Host–guest chemistry plays a crucial role in nature and is closely related to the origin of life [1] , [2] , [3] . It has also allowed for critical advances in environmental science, drug delivery, chemical industry and sensing, among numerous other applications [4] , [5] , [6] , [7] . Macrocycles [8] , such as crown ethers [9] , cyclodextrins [10] , calixarenes [11] , cucurbiturils [12] , and pillararenes [13] , have been central to progress in host–guest chemistry and have permitted seminal advances in molecular recognition [14] , separations [15] , supramolecular materials development [16] and nanotechnology [17] . On the other hand, metal–organic frameworks (MOFs) [18] , [19] , [20] —a class of crystalline framework materials composed of organic struts and inorganic nodes—have been extensively explored for inter alia gas storage [21] , [22] , [23] , water capture [24] , [25] , and catalysis [26] . Not surprisingly, efforts have thus been made to incorporate macrocyclic subunits into MOFs [27] , [28] , [29] . In principle, the resulting systems offer several prospective advantages, including: (1) enhanced regulation of the pore structures allowing for a fine-tuning of the molecular recognition and separation capabilities; (2) better accessibility to active recognition sites; (3) efficient diffusion of guest molecules; (4) clearer insights into structure–property relationships since each recognition site is isolated and amenable to independent study [27] . Unfortunately, crystalline frameworks incorporating well-defined flexible macrocyclic subunits remain challenging to prepare and difficult to characterize [30] . For example, although pillararene-based MOFs have been reported, their structural details remain recondite because rotations of the flexible pillararene subunits can lead to disorder within what are presumably overall periodic frameworks [31] ,\ [32] . Herein, we report a set of pillar[5]arene-containing MOFs denoted as MeP5-MOF-1, MeP5-MOF-2, MeP5-MOF-3 , and MeP5-MOF-4 (Fig. 1a, b ) via the so-called pillar-layer strategy [33] , [34] , [35] , [36] . In these systems, the pillar[5]arene-based MeP5BPy and MeP5BPPy subunits act as ligands for the zinc nodes and may be regarded as macrocycle-bearing struts, while the tetraphenylethylene (TPE) derivatives H 4 TPPE and H 4 TPE also complex the zinc centers and act as layers. As detailed below, single crystal X-ray diffraction (SCXRD) studies of the resulting pillar[5]arene-containing MOFs revealed network interpenetration in the case of MeP5-MOF-2 . This interpenetration restricted the rotation of pillar[5]arene units within the frameworks and allowed the pillar[5]arene subunits to be resolved with atomic resolution. Two prototypical guests, paraquat ( PQT ) and 1,2,4,5-tetracyanobenzene ( TCN ), were tested as guests for MeP5-MOF-1 and MeP5-MOF-2 . Compared with Model-MOF-1 , a MOF lacking an incorporated pillar[5]arene, MeP5-MOF-1 , and MeP5-MOF-2 displayed enhanced guest uptake. These two pillar[5]arene-bearing MOFs allowed for the effective removal of pyridine ( Py ) from toluene ( Tol ) with the toluene purity level up to 99.9% being reached rapidly. The observed selectivity is rationalized on the basis of single crystal structure analyses. Fig. 1: Design and synthesis of pillar[5]arene-based MOFs. a Cartoon representations and chemical structures of ligands and pillar[5]arene-based MOFs: MeP5BPy, MeP5BPPy, H 4 TPE, H 4 TPPE , zinc node, MeP5-MOF- n ( n = 1, 2, 3, 4). b Schematic representations of the transformation from MeP5-MOF-2 to Py @ MeP5-MOF-2 upon uptake of Py from a 90:10 v / v (87.3:12.7 mole percentage) Tol / Py mixture. Py = pyridine; Tol = toluene. Full size image Synthesis of pillar[5]arene-based struts and MOFs Pillar[5]arene-containing struts MeP5BPy and MeP5BPPy were synthesized according to previous reports [37] , [38] (Supplementary Figs. 1 – 5 ). Single crystal structures confirmed that the lengths of these two struts, as judged by the N···N distances, are 11.41 and 19.71 Å, respectively (Supplementary Figs. 24 – 27 ). On this basis, we considered it likely that MeP5BPy and MeP5BPPy could be applied as struts in the “pillar-layer strategy” MOF preparation strategy pioneered by Kim and Hupp using bipydine struts and zinc carboxylates [33] ,\ [35] ,\ [36] (Supplementary Figs. 6 – 17 ). In fact, by applying this strategy using MeP5BPy and MeP5BPPy in conjunction with H 4 TPPE and H 4 TPE it proved possible to prepare MeP5-MOF-1, MeP5-MOF-2, MeP5-MOF-3 , and MeP5-MOF-4 and obtain single crystals suitable for SCXRD analyses. Two model MOFs, Model-MOF-1 and MeModel-MOF-1 , lacking incorporated pillar[5]arene units were also prepared using 1,4-di(4-pyridyl)benzene ( PBPy ) and 4,4’-(2,5-dimethoxy-1,4-phenylene)dipyridine ( MePBPy ) as the struts. Structural determination of pillar[5]arene-based MOFs Proton nuclear magnetic resonance ( 1 H NMR) spectroscopy was used to confirm the presence of the pillar[5]arene struts and TPE carboxylate layers. Taking MeP5-MOF-1 as an example, signals corresponding to H a−f of MeP5BPy and H g−j of H 4 TPPE were seen in the 1 H NMR spectrum (Supplementary Fig. 18 ). The peak integrations were found to match those expected for the structure as well as the mixture of ligands before complexation and after the MeP5-MOF-1 was subject to digestion (treatment with DMSO- d 6 /DCl (100:1 v / v ) and subjecting to ultrasonication to give a transparent solution). Similar results were obtained for Model-MOF-1, MeModel-MOF-1, MeP5-MOF-2, MeP5-MOF-3 , and MeP5-MOF-4 (Supplementary Figs. 19 – 23 ). Further support for the assigned structures came from SCXRD analyses (Supplementary Data 1 ) as discussed below. In the case of MeP5-MOF-1 , the SCXRD analysis revealed a structure that is formulated as [Zn 2 ( MeP5BPy )( TPPE )], which consists of paddlewheel dinuclear Zn 2 (COO) 4 secondary building units (SBUs) bound to carboxylate and pyridine linkers (Supplementary Figs. 28 , 29 ). Each TPPE is coordinated to four Zn 2 nodes to form two-dimensional layers. These layers are joined together by MeP5BPy to form a non-interpenetrated fsc- type framework (Fig. 2a ). The experimental powder X-ray diffraction (PXRD) pattern for MeP5-MOF-1 was similar to that simulated from the SCXRD structure, confirming the phase purity and crystallinity (Supplementary Fig. 66 ). It is worth noting that only the non-pillar[5]arene backbone is observed in the crystal structure of MeP5-MOF-1 . Presumably, this reflects the fact that dynamics of the pillar[5]arene units preclude their being located precisely within the overall framework. Given this absence of direct observation, a structural model, MeP5-MOF-1a , with the pillar[5]arene units shown was constructed (Fig. 2a and Supplementary Figs. 30 , 31 ). The experimental SCXRD data for MeP5-MOF-1 was used as the starting point for constructing this model. The PXRD pattern simulated from the calculated structure of MeP5-MOF-1a proved consistent with that of an as-synthesized MeP5-MOF-1 sample (Supplementary Fig. 32 ). Fig. 2: Structures of MeP5-MOF-1, Model-MOF-1, and MeModel-MOF-1. a Capped-stick representation of structural model MeP5-MOF-1a of MeP5-MOF-1 . Here the backbone of MeP5-MOF-1 was determined by SCXRD, while the pillar[5]arene units are the results of structural model. b Cartoon representation of Model-MOF-1 or MeModel-MOF-1 . c – f Capped-stick representations of single crystal structures of Model-MOF-1 and MeModel-MOF-1 . The TPE ligands are blue, pillared struts are orange, zinc nodes are white, hydrogen atoms and solvent molecules have been omitted for clarity. Full size image Single crystals of the control MOFs, Model-MOF-1 and MeModel-MOF-1 , lacking incorporated pillar[5]arenes were also obtained. The resulting structures revealed that Model-MOF-1 and MeModel-MOF-1 are comprised of [Zn 2 ( PBPy )( TPPE )](DMF) 2 and [Zn 2 ( MePBPy )( TPPE )](DMA) 2 entities. As above, 1 H NMR spectral analysis confirmed the presence of the expected constituent ligands in both Model-MOF-1 and MeModel-MOF-1 (Supplementary Figs. 19 , 20 ). The PXRD patterns of the as-synthesized samples also provided support for the purity and crystallinity of these materials (Supplementary Figs. 67 , 68 ). Of interest is that the crystal structures of Model-MOF-1 and MeModel-MOF-1 revealed two-fold interpenetrated polymeric frameworks. This stands in contrast to what was seen for MeP5-MOF-1 , a framework characterized by a non-interpenetrated structure as noted above. This disparity provides support for the suggestion that the presence or absence of incorporated pillar[5]arene units can control whether or not an interpenetrated MOF structure is obtained (Fig. 2b–f and Supplementary Figs. 33 – 36 ). The observation of interpenetrated structures in the case of Model-MOF-1 and MeModel-MOF-1 provided a motivation to analyze in detail the other MOFs prepared in the context of the present study. A further incentive was to explore whether it would be possible to obtain a structure wherein the incorporated pillar[5]arenes could be located unambiguously. Doing so would address a recognized need since in most reported receptor-incorporated MOFs the flexible macrocycles cannot be located, presumably on account rotation-based disorder as inferred in the case of MeP5-MOF-1 [27] , [31] ,\ [32] ,\ [39] ,\ [40] . Single crystals of MeP5-MOF-2 were obtained via a solvo-thermal procedure, wherein strut MeP5BPPy was combined with 2 equivalent of H 4 TPPE and 2 equivalent of Zn(NO 3 ) 2 . 6H 2 O in DMF (Supplementary Fig. 9 ). Acetic acid was added as a modulator. The crystal structure of MeP5-MOF-2 (Fig. 3a ) revealed that it contains extended pillared struts and is composed of [Zn 2 ( MeP5BPPy )( TPPE )] entities. As true for MeP5-MOF-1, MeP5-MOF-2 possesses a “pillar-layer” structure. However, in contrast to MeP5-MOF-1, MeP5-MOF-2 contains two-fold interpenetrated networks. Moreover, the pillar[5]arene units in MeP5-MOF-2 could be resolved by SCXRD (Fig. 3b and Supplementary Figs. 37 – 42 ). Here, in order to distinguish the dynamics of the pillar[5]arene units in MeP5-MOF-1 and MeP5-MOF-2 , the number of pillar[5]arene units in a 1 nm 3 volume element within the single crystal structures were calculated for both systems [40] . 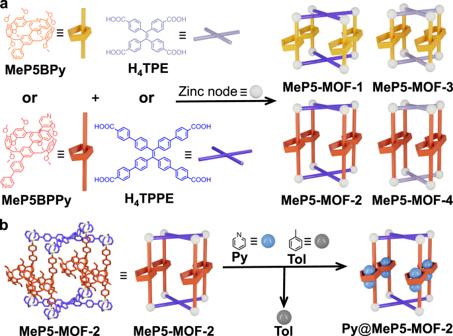Fig. 1: Design and synthesis of pillar[5]arene-based MOFs. aCartoon representations and chemical structures of ligands and pillar[5]arene-based MOFs:MeP5BPy,MeP5BPPy,H4TPE,H4TPPE, zinc node,MeP5-MOF-n(n= 1, 2, 3, 4).bSchematic representations of the transformation fromMeP5-MOF-2toPy@MeP5-MOF-2upon uptake ofPyfrom a 90:10v/v(87.3:12.7 mole percentage)Tol/Pymixture.Py= pyridine;Tol= toluene. Compared with what was seen for single crystal structures of the struts MeP5BPy and MeP5BPPy (0.80 and 0.76 pillar[5]arene units per 1 nm 3 volume element, respectively; Supplementary Table 17 ), MeP5-MOF-1 contains only 0.16 pillar[5]arene units per 1 nm 3 volume element while the corresponding value of MeP5-MOF-2 is 0.23. This low density reflects empty space around the pillar[5]arene and makes both MeP5-MOF-1 and MeP5-MOF-2 dynamic with the latter system less so (Supplementary Figs. 56 – 59 ). Calculations regarding the ability of the pillar[5]arene units to rotate in MeP5-MOF-1 and MeP5-MOF-2 were also carried out. The results revealed that the pillar[5]arene units in MeP5-MOF-1 could rotate 45° along the struts at a minimum potential energy point after optimization. The corresponding value was 10° in MeP5-MOF-2 , which leads us to suggest that the pillar[5]arene units in MeP5-MOF-1 are more flexible than those in MeP5-MOF-2 (Supplementary Figs. 60 , 61 ). Fig. 3: Structures of MeP5-MOF-2, pS -MeP5-MOF-2, and pR -MeP5-MOF-2. a – i Single crystal structures shown in capped-stick form and cartoon representations of MeP5-MOF-2, pS - MeP5-MOF-2 , and pR - MeP5-MOF-2 . The TPE ligands are blue, pillared struts are red, zinc nodes are white, and hydrogen atoms have been omitted for clarity. Full size image SCXRD data of MeP5-MOF-1 were collected at 105 K in an effort to ascertain whether a lower temperature would limit the dynamics of the pillar[5]arene units within the framework. From the single crystal structure of MeP5-MOF-1 , the pillar[5]arene units could still not be visually characterized even at 105 K (Supplementary Figs. 62 , 63 ). Therefore, we ascribe our ability to observe the pillar[5]arene units in MeP5-MOF-2 to the fact that they occupy the internal voids of the frameworks in a pairwise stacked manner, which presumably limits their motion. Each pair consists of MeP5BPPy units in their respective pS and pR conformations (Fig. 3c ). The experimental PXRD pattern also provided support for the purity and crystallinity of the MeP5-MOF-2 sample (Supplementary Fig. 69 ). In order to explore the influence of planar chirality of the pillar[5]arene units in stabilizing the observed rigid MeP5-MOF-2 framework, pre-resolution of racemic - MeP5BPPy was performed. Two enantiomers pS - MeP5BPPy and pR - MeP5BPPy (Supplementary Figs. 45 – 47 ) were separated and used to fabricate the corresponding chiral MOFs, pS - MeP5-MOF-2 and pR - MeP5-MOF-2 (Supplementary Figs. 48 – 51 ). Single crystals of both species were obtained. The Flack parameters for pS - MeP5-MOF-2 and pR - MeP5-MOF-2 were found to be 0.28(2) and 0.26(3). These values lead us to conclude that the absolute structures of these species could not be fully determined, probably due to the partial conformational interconversion between the pS/pR - MeP5 congeners during the preparation of pS/pR - MeP5-MOF-2 (Supplementary Tables 9 , 10 ) [41] , [42] . As true for racemic - MeP5-MOF-2 , both pS - MeP5-MOF-2 and pR - MeP5-MOF-2 consisted of two-fold interpenetrated frameworks. However, the pillar[5]arene struts are oriented toward the layers; in contrast, those of racemic - MeP5-MOF-2 are perpendicular (Fig. 3d–i ). Compared to racemic - MeP5-MOF-2 , the simulated PXRD patterns of pS - and pR - MeP5-MOF-2 from the SCXRD analysis also revealed changes, as would be expected given the differences in the internal spatial arrangement of the constituent pillar[5]arene units (Supplementary Fig. 70 ). When the TPE ligand was changed from H 4 TPPE to H 4 TPE , pillar[5]arene-containing MOFs MeP5-MOF-3 and MeP5-MOF-4 were obtained from MeP5BPy and MeP5BPPy , respectively. As true for MeP5-MOF-1 (and other macrocycle-incorporating systems), the pillar[5]arene units on the struts of MeP5-MOF-3 and MeP5-MOF-4 still could not be located because of disorder (Supplementary Figs. 52 – 55 ). Nevertheless, the experimental PXRD patterns confirmed the phase purity and crystallinity of these two systems (Supplementary Figs. 71 , 72 ). Taken in concert, the studies of MeP5-MOF- n ( n = 1–4) provide support for the intuitively appealing conclusion that frameworks containing struts with incorporated pillar[5]arene units need to limit the dynamics of the flexible macrocycle moiety sufficiently if the macrocycles are to be visualized effectively by SCXRD. Supramolecular recognition of pillar[5]arene-based MOFs for PQT and TCN The clear structural differences between MeP5-MOF-1 and MeP5-MOF-2 (open and interpenetrated) led us to explore their molecular recognition features. Two substrates, namely PQT and TCN , that are known to be bound by pillar[5]arenes [43] ,\ [44] , were chosen as guests for these studies. Fluorescence spectroscopic titration experiments in acetone were performed to determine the association constants and binding stoichiometries between the pillar[5]arenes and guests (Supplementary Figs. 73 – 88 ). On this basis, association constants ( K a ) of 55 ± 1 M –1 , 41 ± 1 M –1 , 53 ± 1 M –1 , and 36 ± 1 M –1 were calculated for PQT @ MeP5BPy, PQT @ MeP5BPPy, TCN @ MeP5BPy , and TCN @ MeP5BPPy , respectively. A 1:1 binding stoichiometry was inferred in all four cases. The solid-state recognition features were also explored. Initially, crystals of MeP5-MOF-1 exhibited a pale-yellow color but changed to dark yellow after uptake of PQT (Fig. 4a, b ). Presumably, this darkening reflects charge transfer interactions between the pillar[5]arene units and the guests. MeP5-MOF-2 also underwent a color change upon exposure to PQT . In contrast, almost no color change was seen for the control, Model-MOF-1 , under otherwise identical conditions (Supplementary Figs. 89 – 91 ). The extent of uptake was determined by calculating the mole ratios of the guests to the struts using the integrated intensities of the corresponding 1 H NMR signals. The 1 H NMR spectra of MeP5-MOF-1, MeP5-MOF-2 , and Model-MOF-1 after uptake of PQT and digestion in DMSO- d 6 /DCl (100:1 v / v ) revealed that the mole ratios of guests to struts were about 0.48, 0.35, and 0.11 (Fig. 4e and Supplementary Figs. 97 – 99 ) for these three MOFs, respectively. Fig. 4: Supramolecular recognition studies of MeP5-MOF-1 and MeP5-MOF-2 with PQT and TCN. Optical microscopy images of MeP5-MOF-1 : a before uptake of PQT ; b after uptake of PQT ; c before uptake of TCN ; d after uptake of TCN . Scale bars, 200 μm. The mole ratios of PQT ( e ) and TCN ( f ) to struts in MeP5-MOF-1, MeP5-MOF-2 , and Model-MOF-1 , as inferred from 1 H NMR spectral studies of these MOFs after guest uptake in acetone. g – i PXRD patterns of single crystalline samples of MeP5-MOF-1, MeP5-MOF-2 , and Model-MOF-1 : I before guest uptake; II after uptake of PQT ; III after uptake of TCN . Source data of g – i are provided as a Source data file. Full size image In the case of TCN , crystalline MeP5-MOF-1 and MeP5-MOF-2 changed from yellow to red (Fig. 4c, d ). This observation was taken as evidence of uptake and the formation of complexes characterized by strong charge transfer interactions between the pillar[5]arene units and the TCN guests within the frameworks. In contrast, little change in color was observed in the case of Model-MOF-1 (Supplementary Figs. 92 – 94 ). Based on analyses analogous to those carried out in the case of PQT , the TCN uptake by MeP5-MOF-1, MeP5-MOF-2 , and Model-MOF-1 was about 0.49, 0.46, and 0.08, respectively (Fig. 4f and Supplementary Figs. 100 – 102 ). PXRD patterns of MeP5-MOF-1, MeP5-MOF-2 , and Model-MOF-1 after uptake of guests revealed evidence for a change in structure while maintaining crystallinity (Fig. 4g–i ). Overall, MeP5-MOF-1 displayed a somewhat higher level of uptake than MeP5-MOF-2 , which in turn displayed more effective guest uptake than Model-MOF-1 lacking incorporated pillar[5]arene units. We thus conclude that the pillar[5]arene units incorporated into MOFs play an active role in supramolecular recognition and that guest uptake is not dictated by simple diffusion. Separation of Tol/Py mixtures using pillar[5]arene-based MOFs The potential utility of pillar[5]arene-containing MOFs for separations was tested using Tol and Py . Tol is one of the most important raw materials in the chemical industry [45] . However, Tol is typically contaminated with trace quantities of Py [46] . It is necessary to remove residual Py from Tol to obtain high-quality Tol . This is a challenging separation compounded by the fact that Tol and Py possess similar boiling points (b.p.) ( Tol : 110.60 °C; Py : 115.50 °C; Supplementary Table 18 ). Moreover, an azeotrope (b.p. 110.20 °C) forms under conditions of distillation [47] . To explore whether the present MOFs could provide a useful alternative, an initial solid–liquid experiment was carried out by soaking crystalline MeP5-MOF-1 in single component Tol or Py for two minutes. The crystals were collected by filtration. The relative uptake of Tol or Py was measured by calculating the mole ratios of Tol or Py relative to the struts using NMR spectroscopy. This analysis revealed that MeP5-MOF-1 could capture 0.6 equivalent of Tol and 6.7 equivalents of Py per pillar[5]arene unit (Supplementary Figs. 109 , 110 ). After solid–liquid adsorption, NMR analysis revealed a 90.8% selectivity for Py obtained from a 100 μL of 90:10 v / v (87.3:12.7 mole percentage) Tol / Py mixture using ~20 mg of crystalline MeP5-MOF-1 (Supplementary Fig. 111 ). A separate quantitative analysis was also performed by heating the samples to release the adsorbed guests and monitoring the volatiles using gas chromatography (GC). This study revealed that (1) the samples adsorbed Py with 90.3% selectivity, a finding consistent with the NMR spectroscopic analysis (Supplementary Fig. 112 ) and that (2) the mole percentage of Tol in the above mixture increased to 96.9% from the initial 87.3% value when ~20 mg samples were used (Supplementary Fig. 113 ). The mole percentage of Tol further increased to 99.9% after the product of the initial separation was treated with another ~20 mg of fresh samples (Supplementary Fig. 114 ). NMR spectroscopic analyses confirmed that roughly 77% of the adsorbed guests in MeP5-MOF-1 could be removed by washing with acetone five times in succession (Supplementary Fig. 115 ). An analogous study was carried out starting with a 99:1 v / v Tol / Py mixture. In this case, the GC analysis revealed that the mole percentage of Tol increased from 98.7% to 99.9% (Supplementary Fig. 116 ). PXRD analyses showed that MeP5-MOF-1 changed its arrangement after guest uptake; presumably, this change reflects the dynamic nature of the framework (Supplementary Fig. 117 ). MeP5-MOF-2 was also tested for its ability to separate Tol / Py mixtures. In this case, initial NMR spectral tests confirmed that MeP5-MOF-2 can accommodate 2.8 equivalents of Tol and 2.6 equivalents of Py per pillar[5]arene unit in single component experiments (Supplementary Figs. 118 , 119 ). A ca. 90.0% selectivity was seen for Py adsorbed from a 100 μL of a 90:10 v / v Tol / Py mixture using ~20 mg sample of crystalline MeP5-MOF-2 (Supplementary Fig. 120 ). GC analyses indicated that the corresponding selectivity of Py was 89.5% which matched what was inferred from the NMR studies (Supplementary Fig. 121 ). The mole percentage of Tol in the resulting mixture increased from 87.3% to 90.5% under these conditions (Supplementary Fig. 122 ). Roughly 87% of the guests in MeP5-MOF-2 could be removed upon washing with acetone five times (Supplementary Fig. 123 ). A PXRD analysis confirmed that, as true for MeP5-MOF-1, MeP5-MOF-2 also changed its arrangement upon uptake of guests (Supplementary Fig. 124 ). An effort was made to obtain diffraction grade single crystals of Py @ MeP5-MOF-2 . Unfortunately, no suitable crystals could be obtained, perhaps as the result of the disordered nature of the Py molecules within the frameworks. Given this, single crystals of Py in 1,4-diethoxypillar[5]arene ( P5 ) were grown by dissolving powdered P5 in Py and allowing to evaporate at room temperature for about one week. The resulting crystal structure revealed that one pillar[5]arene molecule can accommodate two Py molecules within its cavity (Fig. 5a ). Based on the metric parameters, Py binding is driven by [C−H … O] and [C−H … π] interactions ([C … O] distances (Å), [H … O] distances (Å) and [C–H … O] angles (deg) of [C–H … O] hydrogen bonds: 3.42, 2.54, 154.88; 3.42, 2.54, 154.88. [C–H … π] distances (Å) and angles (deg): 3.00, 158.34; 3.07, 158.76. Supplementary Figs. 125 – 127 ). Fig. 5: Structures of (Py) 2 @P5, Py@MeP5-MOF-2, and Tol@MeP5-MOF-2. Illustrated structures of a ( Py ) 2 @ P5 , b , c Py @ MeP5-MOF-2 , and d , e Tol @ MeP5-MOF-2 . The occupancy of Tol in MeP5-MOF-2 is 0.5. Here ( a ), ( d ), and ( e ) are views of single crystal structures, while the Py molecules in ( b ) and ( c ) are models based on the single crystal structure of MeP5-MOF-2 and ( Py ) 2 @ P5 . TPE ligands are blue, pillared struts are red, zinc nodes are white. Hydrogen atoms have been omitted for clarity. Py and Tol are shown in the spacefilling form and color coded by element. Full size image To predict the preferred location of Py molecules within the present MOF frameworks, we carried out sorption module of location simulations based on the single crystal structures of MeP5-MOF-2 and ( Py ) 2 @ P5 (Supplementary Figs. 128 – 130 ). These simulations revealed that the adsorbed Py molecules are retained in the pillar[5]arene cavities (Fig. 5b, c ). Single crystals of Tol @ MeP5-MOF-2 were obtained by immersing MeP5-MOF-2 in a solution consisting of DMF and Tol (5:1 v / v ) for a day. An ensuing SCXRD analysis revealed that as compared with MeP5-MOF-2 , the unit cell of Tol @ MeP5-MOF-2 is relatively constrained. Moreover, the Tol molecules are found within the voids between the TPPE layers rather than in the pillar[5]arene cavities (Supplementary Figs. 132 – 134 ). This stands in contrast to what is seen for Py @ P5 . We rationalize this difference in terms of the smaller size of the Py molecules which makes them more likely to be trapped in the pillar[5]arene cavities. We thus suggest that the pillar[5]arene units incorporated into MeP5-MOF-2 endows the system with an ability to capture Py selectively from Py / Tol mixtures through a macrocycle-dependent recognition process and that this effect is enhanced by confinement within a framework (Fig. 5d, e ). The experimental PXRD patterns of crystalline Py @ MeP5-MOF-2 and Tol @ MeP5-MOF-2 do not quite match the corresponding simulated patterns. While not a proof, this disparity could reflect dynamics in the MOF structure (Supplementary Figs. 131 and 135 ). In contrast, no obvious selectivity of contacting with Py or Tol guests was seen in the case of Model-MOF-1 (Supplementary Figs. 136–140 ). A solid–vapor experiment also confirmed that 1,4-dimethoxypillar[5]arene ( MeP5 ) lacks selectivity in adsorbing Py from Tol / Py mixtures (Supplementary Figs. 141 – 145 ). This result is taken as evidence that confinement within a suitable MOF framework improves the selectivity for Py [48] . We thus conclude that a judicious choice of receptor (e.g., pillar[5]arene) and MOF framework (e.g., MeP5-MOF-2 ) allows for the specific removal of Py from Py / Tol mixtures. We further investigated the efficiency of both MeP5-MOF-1 and MeP5-MOF-2 under bulk conditions (~200 mg). Both MeP5-MOF-1 and MeP5-MOF-2 gave similar results with samples (~20 mg for each) tested as adsorbents (Supplementary Figs. 148 – 153 ). The recyclability of the separation process was also tested. Host–guest studies of MeP5-MOF-1 and MeP5-MOF-2 revealed that some guest molecules were still trapped in MeP5-MOF-1 and MeP5-MOF-2 after each cycle according to 1 H NMR spectroscopic analyses. The corresponding PXRD analyses revealed a partial loss in crystallinity in both MeP5-MOF-1 and MeP5-MOF-2 after each cycle of guest uptake (Supplementary Figs. 154 , 155 ). We also investigated the environmental tolerance of MeP5-MOF-1 and MeP5-MOF-2 under various treatment conditions. The porosity of MeP5-MOF-1 and MeP5-MOF-2 was studied through CO 2 and N 2 adsorption/desorption measurements (Supplementary Figs. 156 – 161 ). Experimental CO 2 adsorption/desorption isotherms at 195 K measuring the porosity of activated MeP5-MOF-1 and MeP5-MOF-2 revealed apparent Brunauer-Emmett-Teller (BET) surface areas of 160 m 2 /g and 190 m 2 /g, respectively. These MOFs are non-porous to N 2 as revealed by N 2 sorption experiments at 77 K. The difference between CO 2 and N 2 is ascribed to the fact that these MOFs showed relative strong affinity for CO 2 compared to N 2 according to another related report [49] . TGA studies of MeP5-MOF-1 and MeP5-MOF-2 were performed to investigate their thermal stability. The resultant TGA curves revealed that MeP5-MOF-1 had only a 3.6% weight loss before around 150 °C, which was assigned to solvent loss, and began to decompose at around 350 °C while samples of MeP5-MOF-2 had a 3.9% weight loss before around 150 °C and began to decompose at around 400 °C (Supplementary Figs. 162 – 165 ). After treatment with some specific solvents, the PXRD patterns revealed that MeP5-MOF-1 and MeP5-MOF-2 still maintained their crystallinity (Supplementary Figs. 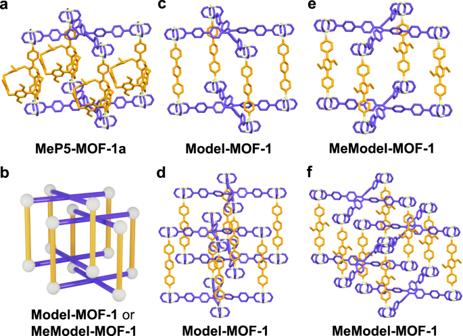Fig. 2: Structures of MeP5-MOF-1, Model-MOF-1, and MeModel-MOF-1. aCapped-stick representation of structural modelMeP5-MOF-1aofMeP5-MOF-1. Here the backbone ofMeP5-MOF-1was determined by SCXRD, while the pillar[5]arene units are the results of structural model.bCartoon representation ofModel-MOF-1orMeModel-MOF-1.c–fCapped-stick representations of single crystal structures ofModel-MOF-1andMeModel-MOF-1. The TPE ligands are blue, pillared struts are orange, zinc nodes are white, hydrogen atoms and solvent molecules have been omitted for clarity. 166 , 167 ). PXRD patterns corresponding to wet and vacuum treatment were also analysed and proved consistent with the notion that these MOFs were dynamic and would lose their partial crystallinity under some conditions (Supplementary Figs. 168 – 171 ). 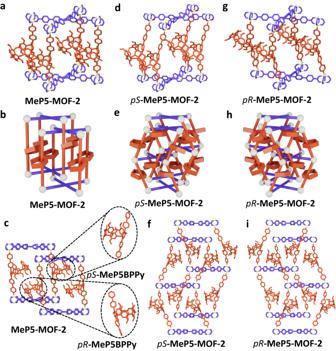Fig. 3: Structures of MeP5-MOF-2,pS-MeP5-MOF-2, andpR-MeP5-MOF-2. a–iSingle crystal structures shown in capped-stick form and cartoon representations ofMeP5-MOF-2,pS-MeP5-MOF-2, andpR-MeP5-MOF-2. The TPE ligands are blue, pillared struts are red, zinc nodes are white, and hydrogen atoms have been omitted for clarity. In conclusion, we have designed and synthesized a set of MOFs incorporating pillar[5]arene motifs. By comparing the structures of these MOFs determined by SCXRD methods we conclude that network interpenetration in the case of MeP5-MOF-2 plays a crucial role in allowing the pillar[5]arene units in the frameworks to be resolved. 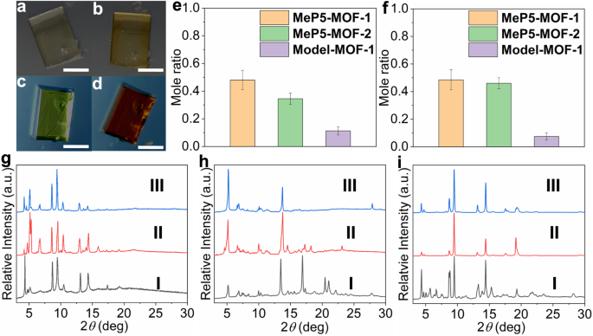Fig. 4: Supramolecular recognition studies of MeP5-MOF-1 and MeP5-MOF-2 with PQT and TCN. Optical microscopy images ofMeP5-MOF-1:abefore uptake ofPQT;bafter uptake ofPQT;cbefore uptake ofTCN;dafter uptake ofTCN. Scale bars, 200 μm. The mole ratios ofPQT(e) andTCN(f) to struts inMeP5-MOF-1,MeP5-MOF-2, andModel-MOF-1, as inferred from1H NMR spectral studies of these MOFs after guest uptake in acetone.g–iPXRD patterns of single crystalline samples ofMeP5-MOF-1,MeP5-MOF-2, andModel-MOF-1:Ibefore guest uptake;IIafter uptake ofPQT;IIIafter uptake ofTCN. Source data ofg–iare provided as a Source data file. 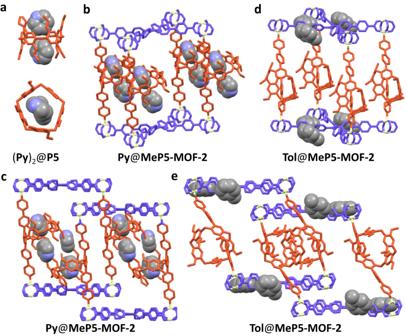Fig. 5: Structures of (Py)2@P5, Py@MeP5-MOF-2, and Tol@MeP5-MOF-2. Illustrated structures ofa(Py)2@P5,b,cPy@MeP5-MOF-2, andd,eTol@MeP5-MOF-2. The occupancy ofTolinMeP5-MOF-2is 0.5. Here (a), (d), and (e) are views of single crystal structures, while thePymolecules in (b) and (c) are models based on the single crystal structure ofMeP5-MOF-2and (Py)2@P5. TPE ligands are blue, pillared struts are red, zinc nodes are white. Hydrogen atoms have been omitted for clarity.PyandTolare shown in the spacefilling form and color coded by element. In other words, we suggest that hindering the rotation of the pillar[5]arene repeating units eliminates their crystallographic disorder within the frameworks. Both MeP5-MOF-1 and MeP5-MOF-2 were found to adsorb PQT and TCN well. In contrast, the pillar[5]arene-free control MOF, Model-MOF-1 , proved relatively ineffective. In addition, both MeP5-MOF-1 and MeP5-MOF-2 could be used to achieve the separation of Py from Tol efficiently and with relative ease. The observation of clear structure–property relationships paves the way for the rational construction of functional framework materials embedded with supramolecular moieties for use in specific recognition and separation application. Single crystal growth Single crystals of MeP5BPPy were grown by dissolving 5.00 mg of dry MeP5BPPy powder in chloroform, heating until all the powder was dissolved and allowing to evaporate about one week. Single crystals of ( Py ) 2 @ P5 were grown by placing 5.00 mg of dry P5 powder in a small vial, adding 1 mL of Py , heating until all the powder was dissolved, and allowing to evaporate at room temperature about one week. Single crystals of Tol @ MeP5-MOF-2 were obtained by immersing MeP5-MOF-2 in a solution consisting of DMF and Tol (5:1 v / v ) for a day. General procedure for preparing single crystals of MOFs Taking MeP5-MOF-1 as an example: A DMF suspension (1.5 mL) of MeP5BPy (8.50 mg, 10.0 μmol), H 4 TPPE (8.10 mg, 10.0 μmol), and Zn(NO 3 ) 2 . 6H 2 O (5.97 mg, 20.0 μmol) was prepared in a small vial. This suspension was sonicated two minutes and then passed through a syringe filter to give a transparent solution, which was sealed, heated at a constant rate of 1 °C min −1 to 90 °C, kept at that temperature for 48 h and cooled to room temperature at a constant cooling rate of 0.2 °C min −1 . Transparent flaxen-colored single crystals of MeP5-MOF-1 suitable for SCXRD were obtained and followed by immersion in 12 mL of acetone for 3 days, with the solvent topped off twice daily.